Perpetual expression of PAMPs necessary for optimal immune control and clearance of a persistent pathogen Pathogen-associated molecular patterns (PAMPs) are known to be fundamental in instigating immune responses, but their role in influencing these responses beyond their initiation is less well understood. Here, using the protozoan parasite Trypanosoma cruzi , which is deficient in strong PAMPs, we demonstrate a requirement for the continuous expression of PAMPs for optimal anti-pathogen immunity. Although co-inoculating with, temporary anchoring of and transgenic expression of exogenous PAMPs all result in enhanced early adaptive immune responses, only the continuous expression of bacterial PAMPs on transgenic T. cruzi sustains these responses, resulting in enhanced pathogen clearance. These findings demonstrate that PAMPs function to potentiate adaptive immune responses well beyond their initiation and may determine the efficiency of control of pathogens capable of long-term persistence. Pathogen-associated molecular patterns (PAMPs) are known to be critical in initiating innate immune responses and in inducing and directing subsequent adaptive immunity [1] , [2] , [3] , [4] . PAMPs are effective indicators of the presence of particular pathogens, in part, because they are unique to classes of pathogens and because they are often required for pathogen survival and thus cannot be altered, suppressed or easily hidden by pathogens. Thus, most of the studies that established the role of PAMPs in innate and adaptive immune responses are based on negating the ability of the host to respond to these molecular patterns [3] , [5] rather than by blocking PAMP expression. However, this has limited our ability to address the relevance of PAMPs to adaptive immunity after its onset. In this work, we make use of the protozoan pathogen Trypanosoma cruzi to evaluate the role of PAMPs in influencing adaptive immunity at and beyond its initiation. T. cruzi is the aetiological agent of Chagas disease, the highest impact human parasitic disease in the Americas. Previous studies have shown that T. cruzi trypomastigotes stimulate a very weak host cell response during invasion [6] and elicit significantly delayed adaptive immune responses [7] , strongly suggesting the relative absence of potent PAMPs on live, invading parasites. Although several endogenous PAMPs have been identified in T. cruzi [8] , [9] , their failure to have an impact on the strength of adaptive immune responses [10] and the ability of certified PAMPs to potentiate immune responses when co-inoculated with T. cruzi [7] have argued against the availability of these putative PAMPs on live T. cruzi [11] and their relevance to anti- T. cruzi immunity. This apparent absence of strong endogenous PAMPs and the genetic pliability of T. cruzi make this pathogen an ideal template for the expression of bona fide PAMPs from other pathogens, and thus for the study of the role of PAMPs beyond the initial phases of immune recognition. In this study, we generate transgenic T. cruzi expressing potent exogenous protein PAMPs and show that this expression not only induces superior innate immune responses but also drives more rapid and persistently stronger adaptive immunity in mice. These studies demonstrate that constitutive expression of PAMPs is instrumental in maintaining a strong adaptive immunity beyond its onset in an infection, leading to better pathogen control and, in some cases, complete parasitological cure. In addition, these findings provide new understanding of how the lack of molecular patterns on the part of some eukaryotic pathogens may fail to incite early immune responses and, thus, provide an opportunity for the establishment of persistent infections. PAMP-transgenic T. cruzi enhances innate immunity We chose to express protein-PAMPs in T. cruzi , as PAMP expression can be stably generated by transgenesis of a single gene, in contrast to polysaccharides or nucleic acid PAMPs, which would require transfer of the entire biosynthetic pathways into T. cruzi . Genes encoding the Salmonella typhimurium flagellin ( fliC ), the ligand for both Toll-like receptor-5 (TLR5; ref. 12 ) and neuronal apoptosis inhibitory protein 5 (NAIP5)/interleukin (IL)-1β-converting enzyme protease-activating factor (ipaf) [13] , and Neisseria meningitidis porin ( porB ), a ligand for TLR1/2 (ref. 14 ), were amplified by PCR and cloned into the pTREX plasmid [15] with a T. cruzi secretory signal peptide from gp72 (ref. 16 ) at their 5′-end ( Supplementary Fig. S1a ). PAMP-transgenic T. cruzi expressing FliC (TcgFliC) or PorB (TcgPorB) were engineered by transfecting these constructs into wild-type (WT), Brazil strain T. cruzi (Tcwt). The signal peptide ensured secretion ( Supplementary Fig. S1b ) of the protein PAMPs expressed by the PAMP-transgenic T. cruzi in epimastigote, trypomastigote and amastigote life stages ( Supplementary Fig. S1c ). Stimulation of TLRs 1/2 or 5 ultimately activates the transcription factors nuclear factor-κB (NF-κB)/activator protein (AP)-1 to promote immunity, primarily by the production of inflammatory cytokines [3] , [17] . NF-κB/AP-1 reporter cell lines exhibited substantially increased levels of NF-κB/AP-1 activation by TcgFliC or TcgPorB live trypomastigotes ( Fig. 1a ) or epimastigote lysates ( Supplementary Fig. S2 ) relative to Tcwt parasites. FliC is also an NAIP5/ipaf ligand that induces IL-1β production in antigen presenting cells (APCs) [13] . FliC-expressing T. cruzi potentiated strong caspase-1 activation ( Fig. 1b ) and modestly enhanced the production of IL1β in TLR5-deficient macrophages ( Fig. 1c,d ), demonstrating that T. cruzi -expressed FliC exhibits both the PAMP-properties of Salmonella flagellin. 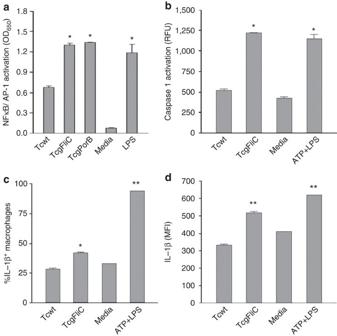Figure 1: PAMP-transgenicT. cruzienhances cellular innate immune responses. (a) NF-κB/AP-1 activation in reporter cells incubated with Tcwt, TcgFliC or TcgPorB trypomastigotes for 12 h. Media orE. coli-derived LPS were used as negative and positive controls, respectively. (b) Caspase-1 activation in (TLR5−) macrophages incubated with Tcwt or TcgFliC trypomastigotes for 12 h. Media or ATP withE. coli-derived LPS served as controls. (c) The proportion of (TLR5−) macrophages producing IL-1β on incubation with Tcwt or TcgFliC trypomastigotes for 18 h. (d) IL-1β mean fluorescence intensity per cell by TLR5−macrophages incubated with Tcwt or TcgFliC trypomastigotes for 18 h. Media or ATP withE. coli-derived LPS served as controls. All data show mean±s.e.m. and are representative of at least three separate experiments. *P≤0.05 or **P≤0.01, as determined by Student’st-test comparing the indicated groups with Tcwt. Figure 1: PAMP-transgenic T. cruzi enhances cellular innate immune responses. ( a ) NF-κB/AP-1 activation in reporter cells incubated with Tcwt, TcgFliC or TcgPorB trypomastigotes for 12 h. Media or E. coli -derived LPS were used as negative and positive controls, respectively. ( b ) Caspase-1 activation in (TLR5 − ) macrophages incubated with Tcwt or TcgFliC trypomastigotes for 12 h. Media or ATP with E. coli -derived LPS served as controls. ( c ) The proportion of (TLR5 − ) macrophages producing IL-1β on incubation with Tcwt or TcgFliC trypomastigotes for 18 h. ( d ) IL-1β mean fluorescence intensity per cell by TLR5 − macrophages incubated with Tcwt or TcgFliC trypomastigotes for 18 h. Media or ATP with E. coli -derived LPS served as controls. All data show mean±s.e.m. and are representative of at least three separate experiments. * P ≤0.05 or ** P ≤0.01, as determined by Student’s t -test comparing the indicated groups with Tcwt. Full size image The innate immune response-inducing activity of PAMP-transgenic T. cruzi trypomastigotes was also evident in IL-12 yet40 reporter mice in which cells expressing IL12/23 p40 subunit also express yellow fluorescent protein (YFP) [18] . Peritoneal exudate macrophages exposed in vitro to PAMP-transgenic T. cruzi produced IL-12 at an increased frequency relative to those exposed to WT T. cruzi ( Fig. 2a ). In addition, TcgFliC and TcgPorB infections of IL-12 yet40 reporter mice resulted in a more rapid and increased infiltration of the IL-12-producing CD11c + CD8α + classical dendritic cells (DCs) into the draining lymph nodes ( Fig. 2b ). TcgFliC infection also altered the lineage bias of the inflammatory cells infiltrating or prevailing at the site of infection, with increased numbers of blood-derived monocytes (CD45 + CD11b + CD11c − Gr-1 int ), macrophages (CD45 + CD11b + CD11c − F4/80 + ), inflammatory DCs (CD45 + CD11b + CD11c hi Gr-1 int ) and other non-classical (CD45 + CD11b + CD11c + CD8α − ) DCs, as compared with WT T. cruzi infection ( Fig. 3a,b ). Classical (CD45 + CD11b − CD11c + CD8α + ) DCs remained undetectable at the site of infection in either case. TcgFliC infection was also associated with enhanced recruitment of IL-12-producing monocytes ( Fig. 3a ) to the site of infection. The innate immune-enhancing effect of PAMP transgenesis was also evident systemically with considerably higher serum levels of IL-12 and tumour necrosis factor-α (TNFα), as compared with Tcwt infection ( Fig ). 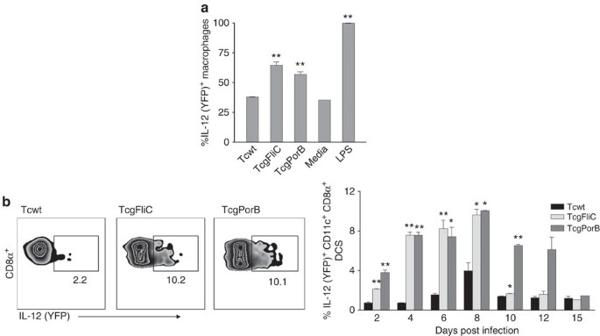Figure 2: PAMP-transgenicT. cruziinduces higher frequencies of IL-12-producing APCs (a) The proportion of peritoneal exudate macrophages with induced IL-12 (YFP) on incubation with Tcwt, TcgFliC or TcgPorB trypomastigotes for 18 h. Media orE. coli-derived LPS served as controls. Data presented as mean±s.e.m. and are representative of three separate experiments. (b) IL-12-producing (CD11c+CD8α+) classical DC (cDC) recruitment into the draining lymph nodes on Tcwt, TcgFliC or TcgPorB infection of IL-12yet40mice. Flow plots show representative data from 6 dpi, with the numbers in the inset indicating the percentage of IL-12-producing cDCs. Right panel shows the kinetics of IL-12+(CD11c+CD8α+) cDC recruitment. Data are represented as mean±s.e.m. from one of three separate experiments, with at least three mice per group. *P≤0.05 or **P≤0.01, as determined by Student’st-test comparing the indicated groups with Tcwt (a), at the corresponding time points (b). Figure 2: PAMP-transgenic T. cruzi induces higher frequencies of IL-12-producing APCs ( a ) The proportion of peritoneal exudate macrophages with induced IL-12 (YFP) on incubation with Tcwt, TcgFliC or TcgPorB trypomastigotes for 18 h. Media or E. coli -derived LPS served as controls. Data presented as mean±s.e.m. and are representative of three separate experiments. ( b ) IL-12-producing (CD11c + CD8α + ) classical DC (cDC) recruitment into the draining lymph nodes on Tcwt, TcgFliC or TcgPorB infection of IL-12 yet40 mice. Flow plots show representative data from 6 dpi, with the numbers in the inset indicating the percentage of IL-12-producing cDCs. Right panel shows the kinetics of IL-12 + (CD11c + CD8α + ) cDC recruitment. Data are represented as mean±s.e.m. from one of three separate experiments, with at least three mice per group. * P ≤0.05 or ** P ≤0.01, as determined by Student’s t -test comparing the indicated groups with Tcwt ( a ), at the corresponding time points ( b ). 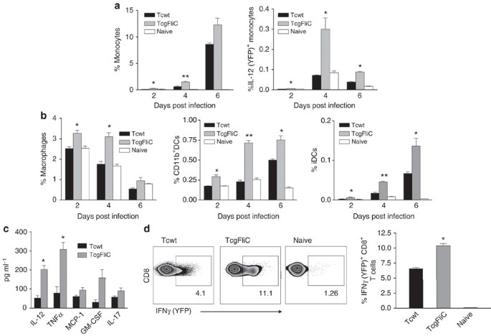Figure 3: PAMP transgenesis inT. cruzienhances the systemic innate immune responses. (a) The proportion of blood-derived monocytes and their IL-12-producing subset at the site (s.c) of Tcwt or TcgFliC infection in IL-12yet40mice at various time points post infection. Naive mice were inoculated with media alone. (b) The proportion of resident macrophages, CD11b+DCs or inflammatory DCs (iDCs) at the site of Tcwt or TcgFliC infection in IL-12yet40mice at various time points post infection. Naive mice were inoculated with media alone. (c) Serum levels of various cytokines in C57Bl/6 mice infected with Tcwt or TcgFliC, 4 dpi. (d) Percentage of CD8+T cells producing IFNγ in the draining lymph nodes with Tcwt- or TcgFliC-infected (foot pad) Yeti mice, 6 dpi. Representative flow plots with the numbers in the inset indicating the percentage of IFNγ-producing CD8+T cells. All data represented as mean±s.e.m. from one of three separate experiments with three to six mice per group. *P≤0.05 or *P≤0.01, as determined by Student’st-test comparing the indicated groups with Tcwt (c,d), at the corresponding time points (a,b). Full size image Figure 3: PAMP transgenesis in T. cruzi enhances the systemic innate immune responses. ( a ) The proportion of blood-derived monocytes and their IL-12-producing subset at the site (s.c) of Tcwt or TcgFliC infection in IL-12 yet40 mice at various time points post infection. Naive mice were inoculated with media alone. ( b ) The proportion of resident macrophages, CD11b + DCs or inflammatory DCs (iDCs) at the site of Tcwt or TcgFliC infection in IL-12 yet40 mice at various time points post infection. Naive mice were inoculated with media alone. ( c ) Serum levels of various cytokines in C57Bl/6 mice infected with Tcwt or TcgFliC, 4 dpi. ( d ) Percentage of CD8 + T cells producing IFNγ in the draining lymph nodes with Tcwt- or TcgFliC-infected (foot pad) Yeti mice, 6 dpi. Representative flow plots with the numbers in the inset indicating the percentage of IFNγ-producing CD8 + T cells. All data represented as mean±s.e.m. from one of three separate experiments with three to six mice per group. * P ≤0.05 or * P ≤0.01, as determined by Student’s t -test comparing the indicated groups with Tcwt ( c , d ), at the corresponding time points ( a , b ). Full size image Interferon-γ (IFNγ) produced by naive CD8 + T cells in a T-cell receptor-independent, IL-12-mediated manner early in the infection seems to serve vital functions in the initial immune responses to a number of pathogens [19] , [20] . To measure the level of IFNγ induced early in response to T. cruzi infection, we used the IFNγ reporter (Yeti) mice, wherein cells expressing IFNγ concurrently express enhanced YFP [21] . At time points when T. cruzi -specific CD8 + T cells are not yet detectable [7] , we observed significantly higher proportions of IFNγ + CD8 + T cells in the draining lymph nodes with TcgFliC infection compared with that with Tcwt ( Fig. 3d ). Taken together, these results indicate that the expression of bacterial PAMPs in T. cruzi markedly enhances innate immune activation both in vitro and in vivo . PAMP-transgenic T. cruzi enhances adaptive immunity A robust T. cruzi -specific CD8 + T-cell response is crucial for the control of T. cruzi infection in mice [22] , [23] , [24] and we have previously shown that the CD8 + T-cell response to T. cruzi in C57BL/6 mice is dominated by cells specific for peptides encoded by the trans -sialidase gene family [25] . Hence, we can use TSKb20 + CD8 + T cells as a surrogate for the total CD8 + T-cell response mounted against T. cruzi , and track this response using the TSKb20/K b tetramers [25] . Mice infected with PAMP-transgenic T. cruzi mounted a more rapid ( Fig. 4a ) and substantially stronger TSKb20 + CD8 + T-cell response that was also maintained at higher levels throughout the infection ( Fig. 4b,c ) relative to WT infected mice. This potentiation of T-cell responses by PAMP-transgenic T. cruzi was also evident in the IFNγ and TNFα production by antigen-experienced CD8 + ( Fig. 4d ) and CD4 + ( Fig. 4e ) T cells. Infection with PAMP-transgenic T. cruzi also elicited higher serum levels of T. cruzi -specific antibodies compared with infection with Tcwt parasites ( Fig. 4f ). 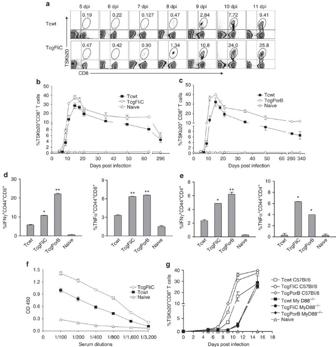Figure 4: PAMP transgenesis inT. cruzienhances the adaptive immune responses generated. (a) Flow plots show early time points post infection in C57BL/6 mice with Tcwt or TcgFliC, with numbers in the inset indicating percentage of TSKb20+CD8+T cells. (b,c) The kinetics of TSKb20+CD8+T-cell frequencies in circulation in TcgFliC (b) and TcgPorB (c) compared with Tcwt infection of C57BL/6 mice. Data represented as mean±s.e.m. from one of six separate experiments, with at least six mice per group. (d,e) The percentage of CD8+(CD44+) (d) or CD4+(CD44+) (e) T cells producing IFNγ (left) or TNFα (right) in response to TSKb20 peptide orT. cruziwhole-cell lysate restimulation, respectively, in Tcwt-, TcgFliC- or TcgPorB-infected C57BL/6 mice, 180 dpi. Data represented as mean±s.e.m. from one of three separate experiments, with three mice per group. (f) Anti-T. cruziantibody titres in sera of mice infected with Tcwt or TcgFliC in C57Bl/6 mice, 30 dpi. Data shown as mean±s.e.m., representing two separate experiments, with three mice per group. (g) The kinetics of TSKb20+CD8+T-cell frequency in circulation on Tcwt, TcgFliC or TcgPorB infection of MyD88−/−or C57Bl/6 mice. Data represented as mean±s.e.m from one of three separate experiments, with three to six mice per group. *P≤0.05 or **P≤0.01, as determined by Student’st-test comparing the indicated groups with Tcwt. Figure 4: PAMP transgenesis in T. cruzi enhances the adaptive immune responses generated. ( a ) Flow plots show early time points post infection in C57BL/6 mice with Tcwt or TcgFliC, with numbers in the inset indicating percentage of TSKb20 + CD8 + T cells. ( b , c ) The kinetics of TSKb20 + CD8 + T-cell frequencies in circulation in TcgFliC ( b ) and TcgPorB ( c ) compared with Tcwt infection of C57BL/6 mice. Data represented as mean±s.e.m. from one of six separate experiments, with at least six mice per group. ( d , e ) The percentage of CD8 + (CD44 + ) ( d ) or CD4 + (CD44 + ) ( e ) T cells producing IFNγ (left) or TNFα (right) in response to TSKb20 peptide or T. cruzi whole-cell lysate restimulation, respectively, in Tcwt-, TcgFliC- or TcgPorB-infected C57BL/6 mice, 180 dpi. Data represented as mean±s.e.m. from one of three separate experiments, with three mice per group. ( f ) Anti- T. cruzi antibody titres in sera of mice infected with Tcwt or TcgFliC in C57Bl/6 mice, 30 dpi. Data shown as mean±s.e.m., representing two separate experiments, with three mice per group. ( g ) The kinetics of TSKb20 + CD8 + T-cell frequency in circulation on Tcwt, TcgFliC or TcgPorB infection of MyD88 −/− or C57Bl/6 mice. Data represented as mean±s.e.m from one of three separate experiments, with three to six mice per group. * P ≤0.05 or ** P ≤0.01, as determined by Student’s t -test comparing the indicated groups with Tcwt. Full size image To reaffirm that the enhanced adaptive immune responses observed with PAMP transgenesis in T. cruzi were indeed dependent on signalling through pattern recognition receptors (PRRs) targeted by the transgenic PAMPs, we infected MyD88 −/− mice that are deficient in the primary adaptor for multiple TLRs and are unresponsive to TLR5, TLR1/2 (ref. 3 ) or (IL-1β from) NAIP5/ipaf stimulation [26] . As expected, the T. cruzi -infected MyD88 −/− mice showed a delayed generation of TSKb20-specific T cells relative to WT mice, with the pattern of responses being similar irrespective of the expression or not of the bacterial PAMPs ( Fig. 4g ). This result indicates that the enhanced adaptive immune response to T. cruzi conferred by PAMP transgenesis is a result of increased triggering of host PRRs and the consequential effects downstream of MyD88 signalling. As many pathogens express multiple PAMPs that cooperate to potentiate adaptive immune responses [27] , [28] , we attempted to co-express both FliC and PorB in T. cruzi . Although C57Bl/6 mice infected with TcgFliC-PorB generated a more rapid and stronger TSKb20 + CD8 + T-cell response as compared with Tcwt, this response was not improved on that generated by either PAMP transgenically expressed alone ( Supplementary Fig. S3a ). This outcome may be a result of technical limitation of protein overexpression in this system, as attempts to overexpress multiple other genes in T. cruzi also resulted in a reduced TcgFliC potency and a reduced expression of the second protein (Paraflagellar Rod Protein 4, PAR4; Supplementary Fig. S3b,c ). This result also suggests that the impact of PAMPs on immune responses may be determined by their relative expression levels in a pathogen. Continuous expression of FliC sustains enhanced adaptive immunity A canonical concept in immunology is that strong innate immunity invokes more potent adaptive immune responses [3] , [5] . This concept is supported by many studies demonstrating that codelivery of TLR ligands with antigens or vaccines significantly boosts adaptive immune responses [29] . However, to our knowledge, no studies have directly investigated the impact on adaptive immunity of a transient presence of PAMPS at the initiation of infection, to a continuous expression of PAMPs throughout the course of infection. Given that PAMP transgenesis in T. cruzi not only initiated a more rapid TSKb20 + CD8 + T-cell response in mice but also resulted in a response that was maintained at unusually high levels, we suspected that PAMPs may have a continuous instructive role in maintaining strong adaptive immune responses. To determine the consequences of transient versus continuous expression of PAMPs on adaptive immune responses to T. cruzi , we tethered various PAMPs to T. cruzi using glycosylphosphatidylinositol (GPI) anchors. Initial experiments showed that molecules linked in this manner were readily incorporated into the surface of trypomastigotes of T. cruzi and had a half-life of ~12 h ( Supplementary Fig. S4a ). The signalling potency of FliC delivered by the GPI tether (Tc-GPI-FliC) or by endogenous expression (TcgFliC) was equivalent as indicated by their similar abilities to induce NF-κB/AP-1 activation in reporter cells ( Supplementary Fig. S4b ) or IL-12 production in peritoneal exudate macrophages ( Supplementary Fig. S4c ). In addition, Tc-GPI-FliC, TcgFliC or native FliC co-inoculated with T. cruzi all potentiated similar innate immune responses to T. cruzi in vivo ( Fig. 5a ) and resulted in a nearly identical early TSKb20 + CD8 + T-cell responses ( Fig. 5b ). However, only in the infection with TcgFliC was the TSKb20-specific response maintained above the level of the Tcwt infection into the chronic stage ( Fig. 5b ). The delivery of other individual or combinations of PAMPs with T. cruzi infection by GPI anchors or by co-inoculation, enhanced innate immune responses in mice—in some, it was enhanced much more strongly than that by TcgFliC ( Supplementary Fig. S4d ). However, only infection with the PAMP-transgenic T. cruzi resulted in the long-term maintenance of enhanced adaptive responses ( Supplementary Fig. S4e ). Repeated injection of flagellin, which is known to induce IL-12 production and activate Th1 responses [30] , [31] , failed to maintain the enhanced CD8 + T-cell responses provided by transgenic expression of flagellin ( Supplementary Fig. S4f ). Thus, continued expression of PAMPs acts to maintain stronger adaptive immune responses, exceeding those elicited by transient PRR engagement at the initiation of infection or thereafter. 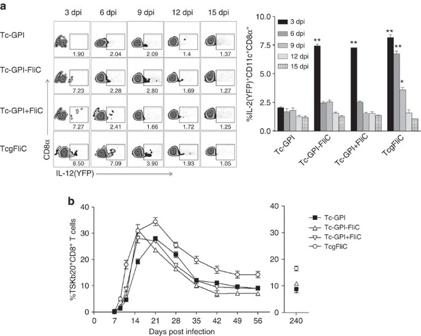Figure 5: Continuous expression of FliC is required to sustain the enhanced adaptive immunity. (a) The proportions of IL-12-producing classical DCs (cDCs) recruited into the draining lymph nodes on various dpi withT. cruzihaving FliC temporarily surface-anchored (Tc-GPI-FliC), co-inoculated with (Tc-GPI+FliC), or constitutively expressed in (TcgFliC), compared with the background strain (Tc-GPI) in IL-12yet40reporter mice. The flow panel shows representative flow plots, with the numbers in the inset indicating the %IL-12+cDCs. Data are represented as mean±s.e.m. from one of three separate experiments, with at least three mice per group per time point. *P≤0.05 or **P≤0.01, as determined by Student’st-test comparing the indicated groups with Tcwt-GPI at the corresponding time points. (b) TSKb20+CD8+T-cell frequency in circulation in Tc-GPI, Tc-GPI-FliC, Tc-GPI+FliC or TcgFliC infection of C57BL/6 mice. Data represented as mean±s.e.m. combining two experiments, with three to six mice per group. Figure 5: Continuous expression of FliC is required to sustain the enhanced adaptive immunity. ( a ) The proportions of IL-12-producing classical DCs (cDCs) recruited into the draining lymph nodes on various dpi with T. cruzi having FliC temporarily surface-anchored (Tc-GPI-FliC), co-inoculated with (Tc-GPI+FliC), or constitutively expressed in (TcgFliC), compared with the background strain (Tc-GPI) in IL-12 yet40 reporter mice. The flow panel shows representative flow plots, with the numbers in the inset indicating the %IL-12 + cDCs. Data are represented as mean±s.e.m. from one of three separate experiments, with at least three mice per group per time point. * P ≤0.05 or ** P ≤0.01, as determined by Student’s t -test comparing the indicated groups with Tcwt-GPI at the corresponding time points. ( b ) TSKb20 + CD8 + T-cell frequency in circulation in Tc-GPI, Tc-GPI-FliC, Tc-GPI+FliC or TcgFliC infection of C57BL/6 mice. Data represented as mean±s.e.m. combining two experiments, with three to six mice per group. Full size image FliC transgenesis boosts immune control of T. cruzi To investigate the impact of the PAMP-induced enhancement of innate and adaptive immune responses on the parasite control during the course of T. cruzi infection, we first monitored the phenotype of T. cruzi -specific CD8 + T cells in these mice. Drug-induced cure of T. cruzi infection results in a gradual shift in the TSKb20 + CD8 + T cells from a predominant T-effector phenotype (CD127 lo ) to a majority T-central memory-like (CD127 hi ) phenotype [22] , accompanied by a decrease in the frequency of CD8 + T cells expressing KLRG1, a marker for repeated antigenic stimulation [22] , [32] . At 296 days post infection (dpi), TcgFliC-infected mice exhibited higher proportions of T-central memory-like phenotype CD127 hi TSKb20 + CD8 + T cells and decreased numbers of KLRG1 + (CD44 + )CD8 + T cells in comparison with mice infected with WT T. cruzi ( Fig. 6a ), suggesting more effective control of the infection with TcgFliC. This supposition was confirmed using quantitative PCR to measure T. cruzi DNA in muscle tissue from these mice ( Supplementary Fig. S5 ). At 400 dpi, T. cruzi DNA was undetectable in mice infected with TcgFliC, but was consistently detected in tissues from Tc-GPI-FliC-, Tc-GPI+FliC- and Tcwt-infected mice ( Fig. 6b ). In contrast, neither changes in the phenotypes of T. cruzi -specific CD8 + T cells nor a decrease in tissue parasite loads were evident in the case of TcgPorB-infected mice, despite their enhanced innate and adaptive immune responses (Supplementary Fig. S6). 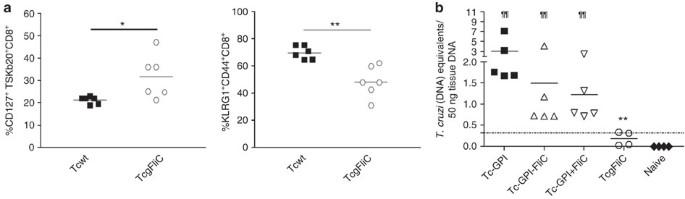Figure 6: FliC transgenesis enhances control ofT. cruziinfection in mice. (a) Frequency of CD8+T cells in circulation having Tcm-like phenotype (CD127hiTSKb20+CD8+(left) and KLRG1loCD44+CD8+(right)), in Tcwt or TcgFliC-infected C57BL/6 mice, 296 dpi. Data represents three separate experiments with three to six mice per group. *P≤0.05 or **P≤0.01, as determined by Student’st-test.(b)T. cruziDNA in skeletal muscle of C57BL/6 mice inoculated with Tcwt, Tc-GPI-FliC, Tc-GPI+FliC or TcgFliC as determined by quantitative real-time PCR, 400 dpi. Horizontal bars represent the mean. Naive mice served as control. The dotted line represents the threshold of detection for the assay. Data are representative of three separate experiments initiated with at least five mice per group. ¶¶ or ** indicatesP≤0.01 comparing the indicated groups with naive or Tcwt-infected mice, respectively, as determined by Student’st-test. Figure 6: FliC transgenesis enhances control of T. cruzi infection in mice. ( a ) Frequency of CD8 + T cells in circulation having Tcm-like phenotype (CD127 hi TSKb20 + CD8 + (left) and KLRG1 lo CD44 + CD8 + (right)), in Tcwt or TcgFliC-infected C57BL/6 mice, 296 dpi. Data represents three separate experiments with three to six mice per group. * P ≤0.05 or ** P ≤0.01, as determined by Student’s t -test. ( b ) T. cruzi DNA in skeletal muscle of C57BL/6 mice inoculated with Tcwt, Tc-GPI-FliC, Tc-GPI+FliC or TcgFliC as determined by quantitative real-time PCR, 400 dpi. Horizontal bars represent the mean. Naive mice served as control. The dotted line represents the threshold of detection for the assay. Data are representative of three separate experiments initiated with at least five mice per group. ¶¶ or ** indicates P ≤0.01 comparing the indicated groups with naive or Tcwt-infected mice, respectively, as determined by Student’s t -test. Full size image We have previously used immunosuppression to reveal otherwise undetectable infection and as a definitive measure of drug-induced cure in T. cruzi infection [22] . One of three TcgFliC-infected mice immunosuppressed with cyclophosphamide exhibited no detectable parasites after immunosuppression, indicating clearance of the infection. The enhanced control of the TcgFliC infection relative to WT T. cruzi infection was neither due to a decrease in virulence of the FliC-transgenic parasites, as IFNγ −/− mice infected with TcgFliC or Tcwt showed similar peripheral blood parasite loads and mortality patterns ( Supplementary Fig. S7 ), nor to immune responses directed at FliC presented as an antigen ( Supplementary Fig. S8 ). Taken together, these data indicate that FliC transgenesis, but not co-inoculation or temporary surface-anchoring, potentiates anti- T. cruzi adaptive immune responses and facilitates control and clearance of T. cruzi infection. One of the key paradigms in immunology is that innate immune mechanisms detect microbial infections through their characteristic PAMPs and trigger the specific antimicrobial host defense responses appropriate to that infection [29] , [33] , [34] . Once initiated, these pathogen-specific (adaptive) immune responses bring about control of the infection and often a long-term specific immunological memory. However, we have very limited knowledge of the role of PAMPs in influencing the adaptive immunity beyond its initiation, in large part because, by their very nature, PAMPS are crucial for pathogen survival and thus cannot be turned off during an infection. In this study, we provide unequivocal evidence that the expression of classical bacterial PAMPS in the protozoan pathogen T. cruzi results in substantially enhanced innate and adaptive immune responses and more efficient pathogen control. These data add to the wealth of information, indicating that T. cruzi has an extremely quiet entry into hosts [6] and a considerably delayed induction of antiparasitic immune responses [7] . Although PAMPs are highly conserved structures that are extremely difficult for pathogens to alter or sacrifice, there is some plasticity in PAMP display. For example, host detection of lipopolysaccharide (LPS) in Porphyromonas gingivalis and Escherichia coli is modulated by differential acylation of lipid A [35] , [36] , whereas Yersinia pestis synthesizes LPS–lipid A, which is a poor TLR4 ligand [37] , and Pseudomonas aeruginosa downregulates its flagellin expression when in airway passages [38] . Although it is unlikely that any pathogen will be able to make all its PAMPs entirely invisible to the immune system, we believe that potential PAMPs could be rendered immunologically inconsequential by concealing or modifying them, without having a significant impact on pathogen biology. Multiple PAMPs (for example, GPI anchors, DNA and glycosylinositol phospholipid (GIPL) ceramide) have been attributed to T. cruzi [8] , [9] but these molecules seem to be relatively insignificant to the downstream immune responses generated, with comparable adaptive immunity in mice that are either responsive or (genetically) unresponsive to these ligands [10] . Perhaps this is not surprising, as these putative PAMPs would be ‘hidden’ from their respective TLRs in live, intact T. cruzi . However, when strong bacterial PAMPs are transgenically expressed and released by T. cruzi , significantly improved innate and adaptive immune responses are generated. Hence, we propose that the failure of T. cruzi to display potent PAMPs may indeed be another example of innate immune evasion employed by pathogens. The observed evasion of innate immune responses may not only be important in delaying the adaptive immune response, thus allowing for firm establishment of the infection, but also may promote the persistence of T. cruzi . In the presence of a bacterial PAMP, T. cruzi infection is better controlled and even completely cleared in some cases. It is to be noted that complete clearance of T. cruzi infection is normally extremely rare. Given the increased level of T. cruzi -specific CD8 + T cells with a Tcm phenotype and the nearly undetectable tissue parasite load in mice infected with PAMP-transgenic T. cruzi , we predict that most of these mice would eventually cure these infections if allowed sufficient time. Importantly, this enhanced control of T. cruzi infection derived from the expression of bacterial PAMPs is not associated with any evidence of increased immunopathology. The relative absence of PAMPs in T. cruzi provided a unique opportunity to study the importance of PAMP expression beyond the early induction of adaptive immune responses. Although there is a wealth of literature demonstrating how the strength of innate immunity determines the potency of adaptive immune responses [33] , [34] , few studies have focused on the impact of innate immune responses on adaptive immunity once an infection is established. When potent bacterial PAMPs were either co-inoculated with, temporarily surface-anchored on or constitutively expressed by the invading T. cruzi , the resulting adaptive immune responses were not only accelerated but also peaked early at levels which were above that seen in mice infected with WT T. cruzi . However, it was only when T. cruzi perpetually expressed the PAMPs that the stronger adaptive immune responses were maintained throughout the course of the infection, eventually leading to a better control of the pathogen and sterile clearance in some cases. It is likely that the locally enhanced inflammatory milieu, coupled with the improved antigen processing and presentation by more highly activated APCs resulting from continuing PAMP exposure [33] , [39] , potentiated the quality, quantity and longevity of T and B cells [40] , [41] , [42] , [43] . Although transgenic expression of FliC and PorB induced similar boosting of immune responses, it was only in the case of TcgFliC that this response corresponded with better parasite control. FliC is distinctive in its ability to induce IL-1β through the intracellular NAIP5/ipaf receptor stimulation, and given that T. cruzi spends the majority of its time in vertebrates within the cytoplasm of host cells that are likely to express the NAIP5/ipaf receptor [44] , it is possible that NAIP5/ipaf–IL-1β activation contributes to enhanced recognition and control of TcgFliC-infected cells. IL-1β levels have also been shown to correlate with CD8 + T-cell abundance in adipose tissues [45] , which incidentally is a major depot for T. cruzi persistence chronically. A possible confounder in the interpretation of our results is that FliC expressed by TcgFliC may act as a target antigen for adaptive immune responses, contributing to the control of FliC-expressing parasites. However, the absence of detectable FliC-specific T cells in TcgFliC-infected mice argues against this possibility. Heterologous expression of bacterial PAMPs in T. cruzi , despite prompting stronger adaptive immune responses, could only marginally (although significantly) accelerate the initial induction of these responses. Hence, the deficiency of effective PAMPs in T. cruzi may be only one of the several factors that contribute to the marked delay in initiation of anti- T. cruzi immune responses. An additional important trigger for induction of adaptive responses is the exposure of damage-associated molecular patterns [46] . Revelation of damage-associated molecular patterns from either host or T. cruzi would not be expected until 4–5 dpi, with the initial round of exit of T. cruzi from infected host cells. This study provides significant new insights into the T. cruzi –host interface and identifies some of the contributing factors for the ability of T. cruzi to persist indefinitely in most hosts, despite the generation of potent immune responses. The contribution of inadequate PAMP expression in the persistence of other pathogens, in particular eukaryotic pathogens that lack many of the classical PAMPs, is worthy of further exploration. Our findings also advance the idea that innate immune responses may have an extended, instructive role on the adaptive immunity, thus having an even more significant part in the effective control of pathogens than was previously appreciated. The inability of classical adjuvants to generate a long-lasting enhancement of T-cell responses has been a hurdle in the development of T-cell-based vaccines [29] . The expression of heterologous PAMPs would be expected to enhance the effectiveness of live vaccines, and periodic or continuous exposure to PAMPs might have therapeutic benefit in persistent infections wherein endogenous PAMPs are inadequate. Mice and infections C57BL/6, B6.IFNγ-knockout (IFNγ −/− ), MyD88 knockout (MyD88 −/− ), B6.IL-12 yet40 reporter (IL-12 yet40 ) and IFNγ reporter (Yeti) mice were purchased from The Jackson Laboratory or bred and maintained in our animal facility under specific pathogen-free conditions to use females of 6–8 weeks old for the experiments. T. cruzi epimastigotes were transfected [16] with pTREX plasmid [15] containing the coding sequence of S. typhimurium flagellin (FliC), N. meningitidis (FAM18 strain) porin (PorB) or T. cruzi PAR4, with or without fusion to an upstream amino-terminal portion of the T. cruzi gp72 or influenza haemagglutinin (HA)-tag, to generate transgenic T. cruzi . All infections were initiated by inoculating vero cell culture passaged-trypomastigote stage T. cruzi , intraperitoneally (10 4 parasites) or subcutaneously in the ear (5 × 10 4 parasites) or in the foot pad (10 4 parasites). Native FliC was inoculated intraperitoneally in mice at 10 μg per animal [31] at 10-day intervals. All animal protocols were approved by the University of Georgia Institutional Animal Care and Use Committee. Reporter cell assays The ability of various T. cruzi strains to induce NF-κB/AP-1 activation by TLR stimulation was assayed using THP1-Blue-CD14 reporter cells (Invivogen), following the manufacturer’s protocol. Live T. cruzi trypomastigotes (10 4 ) were incubated with 2 × 10 6 reporter cells for 9 h at 37 °C/5% CO 2 , and the nuclear translocation of activated NF-κB/AP-1 was determined by colorimetrically quantifying the secreted embryonic alkaline phosphatase. To determine the IL-12 production induced in cells by T. cruzi , 10 5 peritoneal exudate macrophages from IL-12yet40 reporter mice were incubated with 10 3 T. cruzi trypomastigotes for 18 h at 37 °C/5% CO 2 . The proportion of YFP + macrophages was determined by flow cytometry. LPS or media served as controls. Determination of caspase-1 activity Active caspases were detected with FLICA Apoptosis Detection kit (Immunochemistry Technologies) following the manufacturer’s protocol. After 12 h incubation of 2 × 10 4 TcgFliC or Tcwt with 2 × 10 5 RAW blue (TLR5−) mouse macrophages (Invivogen), the latter was incubated with a fluorescent inhibitor peptide specific to caspase-1 (FAM-YVAD-FMK) for 60 min at 37 °C/5% CO 2 . Inhibitors were removed by rinsing; the cells were fixed and then analysed with a florescence plate reader. Western blot and ELISA assay To determine the presence of FliC, TcgFliC lysate [47] or culture (12 h) supernatant were probed with anti-FliC Mab (1:500; Biolegend) by western blotting. Sera collected from C57BL/6 mice infected with various T. cruzi strains 30 dpi were assayed for anti- T. cruzi antibodies by ELISA. To determine the relative concentrations of HA-tagged protein (PAR4-HA) in the trypomastigote stage from various strains of transgenic T. cruzi , serial dilutions of whole-cell lysates were assayed with anti-HA antibody (1:1,000; Roche). A purified HA-tagged protein ( T. cruzi PAR2) expressed in E. coli was used as the standard. Intracellular cytokine staining To measure IL-1β production, 2 × 10 5 RAW blue (TLR5 - ) mouse macrophages (Invivogen) were incubated with 2 × 10 4 TcgFliC trypomastigotes for 18 h. E. coli LPS+ATP or media served as controls. The induced IL-1β in macrophages were determined by staining using the Cytofix/Cytoperm intracellular staining kit (BD Pharmingen) following the manufacturer’s protocol. Similarly, to determine intracellular IFNγ and TNFα production, 1.5 × 10 6 spleen cells from TcgFliC, TcgPorB- or Tcwt-infected, or naive mice were restimulated with T. cruzi peptide TSKb20 (5 μM), T. cruzi whole-cell lysate (10 μg) or FliC, and processed for intracellular cytokine staining. Recombinant ovalbumin protein (ova) or recombinant ovalbumin protein with TSKb20 peptide substituted for SIINFEKL(Ova-TS20) served as a controls. The splenocytes were washed in resuspension buffer (2% BSA, 0.02% azide in PBS) and stained for surface expression of CD4, CD44 and CD8 using anti-CD4 PE (1:100), anti-CD44 FITC (1:400) and anti-CD8 eFluor450 (1:800; BD Pharmingen), respectively. All cells for intracellular cytokine staining were fixed and permeabilized using Cytofix/Cytoperm (BD Pharmingen) on ice for 15 min and washed in PermWash (BD Pharmingen). The cells were then stained with anti-IL-1β PE (1:100; R&D systems), anti-IFNγ APC (1:400) or anti-TNFα PECy7 (1:400; both BD Pharmingen) for 30 min on ice. Cells were washed and fixed in 2% formaldehyde for 20 min at 4 °C, then washed and resuspended in resuspension buffer for flow cytometric analysis. Phenotyping cells by flow cytometry T-cell phenotypes were determined [22] by staining with tetramer–phycoerythrin (TSKb20-PE; ANYKFTLV peptide on H2K b NIH Tetramer Core Facility) and the following: anti-CD62L APC (1:100), anti-CD44 FITC (1:400), anti-CD8 efluor-450 (1:800), anti-CD127 PEcy7 (1:100) and anti-KLRG1 APCcy7 (1:100; all from eBioscience). Anti-CD4 PECy5 (1:200; Invitrogen) and anti-B220 PECy5 (1:200; Invitrogen) staining were used for a dump channel. To determine the phenotypes of cells infiltrating the site of infection, the tissue (ear) was enzymatically digested to dissociate the cells . In the case of draining lymph nodes, the cells were dissociated by gently crushing between the ground edges of glass slides. After FcR (CD16/ 32) block, cell surface markers were used to differentiate several cell lineages [48] . DCs, infiltrating monocytes or resident macrophage subsets were differentiated using the following monoclonal antibody conjugations: CD11c APC (1:100), CD8α efluor450, CD11b APC/eFluor780 (1:800), Gr-1(Ly6C/Ly6G) PerCP/Cy5.5 (1:200), F4/80 PECy7 (1:200) and CD45 PE (1:200; BD Pharmingen, eBioscience or BioLegend). DCs were defined with CD11c, with further differentiation into CD11b − CD8α + classical DCs and CD11b + (F4/80 − ) DCs. Monocytes and immature DCs were defined as CD11b + CD11c − Gr-1 int and CD11b + CD11c + Gr-1 int , respectively [49] . Macrophages were identified as F4/80 + CD11b + CD11c − . IL-12-producing DCs were defined as CD11c + CD8α + (CD11b − ) YFP + in IL-12 yet40 reporter mice as described before [18] . Data are represented as the percentage of each cell type over all the cells derived by enzymatic digestion, representing the total cellularity at the site. IFNγ-producing CD8 T cells in the draining lymph nodes of yeti mice were defined as CD4 − B220 − CD8 + YFP + as described before [50] . At least 5 × 10 5 (blood) or 5 × 10 6 (peripheral tissue/lymph node) cells were acquired per sample using a CyAn flow cytometer (Beckman Coulter) and analysed with FlowJo software (Tree Star). Serum cytokine assay The blood samples were collected from C57Bl/6 mice inoculated with TcgFliC or Tcwt and sera separated to assay for various cytokines using the Q-Plex Mouse Cytokine Screen ELISA (Quansys Biosciences), or for IL-12 alone using eBioscience mouse IL-12p70 flowCytomix, following the manufacturer’s protocol. Luminescence intensity of each sample was measured and the concentration of each cytokine was determined using the Q-View software (Quansys Biosciences) in the former or by flow cytometry for the latter. Temporary anchoring of PAMPs on T. cruzi FSL-biotin GPI anchor with a single biotin F-moiety (FSL-CONJ(1Biotin)-SC2-L1, KODE Biotech Materials Ltd) was used to coat T. cruzi trypomastigotes as per the manufacturer’s protocol. Trypomastigotes (1 × 10 6 ) were incubated with 2 μg of FSL-biotin in 100 μl serum free RPMI 1640 media. After washing to remove the excess FSL-biotin, the parasites were incubated on ice with streptavidin (Sigma), at five times the molar concentration of FSL-biotin (to give Tc-GPI). Excess streptavidin was removed by washing and various biotinylated ligands: FliC-biotin, Pam3CSK4-biotin (Pam3Cys-Ser-(Lys)4-biotin, Invivogen), ODN-biotin (oligodeoxynucleotide-biotin, Invivogen), all at 3 × molar concentration of FSL-biotin, or Pam3CSK4-biotin and ODN-biotin together, each at 1.5 × molar concentration of FSL-biotin, were incubated with the Tc-GPI for 30 min on ice to yield Tc-GPI-FliC, Tc-GPI-Pam3CSK4, Tc-GPI-ODN or Tc-GPI-ODN-Pam3CSK4, respectively. FliC was biotinylated using EZ-link sulpho-NHS-LC Biotinylation kit (Thermo Scientific), following the manufacturer’s protocol. The various PAMP-anchored T. cruzi strains were washed twice with RPMI1640 to remove excess PAMPs, counted, resuspended in complete RPMI 1640 and used for in vitro or in vivo assays. Tc-GPI was used as the control. PAMPs, when co-inoculated with T. cruzi , were used at approximately the same quantities (in w/v) as was used to label T. cruzi above. Real-time PCR The skeletal muscle tissue from mice were analysed by real-time PCR for the presence of T. cruzi (DNA) using the following primer pairs—TCSat30: 5′-GGCGGATCGTTTTCGAG-3′ and TCSat179: 5′-AAGCGGATAGTTCAGGG-3′ (ref. 51 ). Assessment of infectivity and clearance of T. cruzi To assess the infectivity of different strains of T. cruzi , IFNγ −/− mice were inoculated with 10 4 trypomastigotes of TcgFliC or Tcwt strains. Blood was collected from the tail vein at 21 dpi to quantify the number of parasites using a compound light microscope and expressed as the number of live trypomastigotes per 100 ( × 40) fields. Survival was monitored daily. Complete clearance of T. cruzi from infected mice was assessed by real-time PCR amplification of T. cruzi DNA in skeletal muscle obtained following immunosuppression with cyclophosphamide (200 mg kg −1 ; 4 × at 2-day intervals) [22] . Statistical analysis Data are presented as the mean±s.e.m. Statistical analyses compared the groups with a two-tailed Student’s t -test. Only P -values<0.05 were considered statistically significant. How to cite this article: Kurup, S. P. & Tarleton, R. L. Perpetual expression of PAMPs necessary for optimal immune control and clearance of a persistent pathogen. Nat. Commun. 4:2616 doi: 10.1038/ncomms3616 (2013).